Gate-controlled electron transport in coronenes as a bottom-up approach towards graphene transistors Since the discovery [1] of graphene, graphene field effect transistors (FETs) have been widely studied because of their interesting transport properties and potential electronic applications [1] , [2] , [3] . To date, graphene FETs have been fabricated through either mechanical exfoliation of bulk graphite or epitaxial growth on crystal surfaces [2] . Some of these devices that exhibit extremely high carrier mobilities [4] , [5] are desirable for high-speed electronics applications [6] . However, the absence of a bandgap for this material gives rise to very small on/off ratios, which constitutes the main limitation of the device performance [7] . To open up a bandgap in graphene, a top-down approach has been used to cut graphene sheets into nanoribbons with widths below 10 nm [8] . These graphene nanoribbon FETs indeed show much improved on/off ratios, but defects in the graphene ribbons, disorders at the edges, and impurities in the supporting substrate remain as scattering sources that limit the mobilities of these devices. An alternative approach to fabricate graphene nano-FETs is to synthesize graphene molecules, starting from small building blocks. This bottom-up approach has several potential advantages [9] : (1) it allows one to fabricate devices using mass produced and virtually identical molecules; (2) each molecule is defect- and disorder free, and has precisely known number and positions of atoms; (3) the electronic properties can be tuned by adjusting the size and shape of the molecules, resulting in bandgap electronic structures; (4) chemical properties of the molecules can be controlled by introducing side groups; and (5) well-defined molecule–electrode contacts can also be introduced by adding terminal groups to the molecules. To use this approach to fabricate graphene FETs, one faces several technical challenges. The first one is to synthesize large enough graphene molecules, which has been a difficult task of synthesis. The second challenge is to assemble individual molecules into a device, and measure the electron transport in the devices. Finally, one must also be able to provide a third electrode to apply a gate voltage to control the source-drain current. In this study, we synthesized two coronene derivatives, each consisting of 13 aromatic rings arranged into a well-defined honeycomb structure. We determined the conductance of the molecules, studied charge transport in single coronene molecules as a function of electrochemical gate voltage and observed pronounced n-type gating effect in these single coronene devices. The structures of the two studied derivatives of hexa- peri -hexabenzocoronene (HBC) are sketched in Fig. 1 . Each consists of 13 aromatic rings, and has two terminal groups that can bind to electrodes for electrical contacts. The terminal groups in 1 are amines, which have been shown to provide good contact to gold electrodes [10] , [11] . 2 , in contrast, has two thiols as terminal groups, which are separated from the coronene core by additional spacers. In general, nonsubstituted polycyclic aromatic hydrocarbon molecules tend to aggregate by the π–π stacking force. This tendency is minimized by using organic solvents, such as toluene and mesitylene, and by introducing branched side chains to the molecules. Protecting groups on the thiolated linkers were engineered to further reduce aggregation (see Supplementary Scheme S2 : synthetic route of 2 ). Ultraviolet-visible absorption and matrix-assisted laser desorption/ionization–time of flight characteri-zation of solutions containing both 1 and 2 suggest a high chemical stability of the compound with no evidence of aggregation and/or polymerization. We used a scanning tunnelling microscope (STM) configuration to bridge HBC molecules between the gold tip and substrate electrodes, and to measure transport current through the molecules. To effectively apply a gate voltage to control the source-drain current, we used an electrochemical gate with ionic liquid, 1-butyl-3-methylimidazolium hexafluorophosphate, as the gate medium. 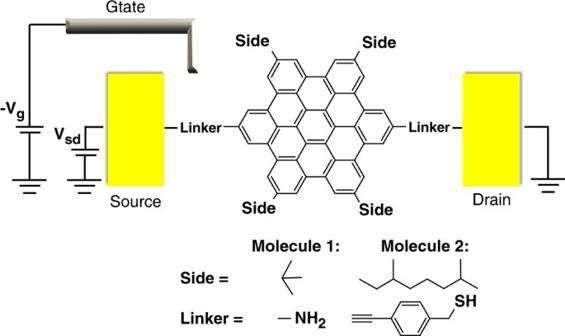Figure 1: Single HBC molecule FET. Two HBC molecules, each consisting of 13 aromatic rings and terminated with two linker groups that can bind to the source and drain electrodes. Molecule1is terminated with two amine groups, and molecule2is terminated with two ethynyl–phenyl–methylene thiol groups. Both of the molecules are substituted with four alkyl side chains for solution-phase processing. Figure 1: Single HBC molecule FET. Two HBC molecules, each consisting of 13 aromatic rings and terminated with two linker groups that can bind to the source and drain electrodes. Molecule 1 is terminated with two amine groups, and molecule 2 is terminated with two ethynyl–phenyl–methylene thiol groups. Both of the molecules are substituted with four alkyl side chains for solution-phase processing. Full size image We first determined the conductance of HBC molecules by using the STM break junction method [12] . The STM tip was first moved into contact with the molecules adsorbed on the substrate, and then pulled away from the substrate, by which a molecule could bridge between the tip and substrate electrodes. The process was repeated quickly for thousands of iterations. 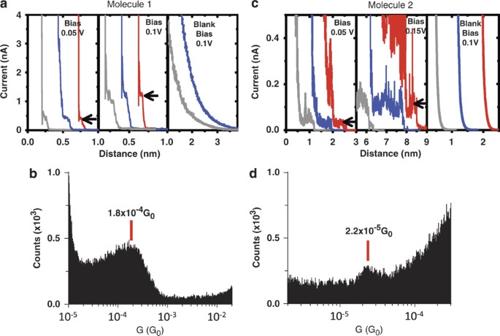Figure 2: Conductance of single HBC molecules. (a) Individual conductance traces of1. Observed plateaus (arrows) are due to the breakdown of molecule–electrode contacts. For comparison, control experiments carried out in the absence of molecules are also shown. (b) Conductance histogram constructed from thousands of individual conductance traces for1. (c) Individual conductance traces of2. (d) Conductance histogram constructed from thousands of individual conductance traces for2. Note that the large counts near the edges on both histogram plots (b,d) are due to background noises. Figure 2a shows several conductance traces recorded during individual pulling processes for 1 , in which the steps pointed by arrows are due to the attachment of an HBC molecule between the tip and substrate electrodes. Statistical analysis of ∼ 1000 individual conductance traces shows a peak near 1.8×10 −4 G 0 , where G 0 =2e 2 /h ( Fig. 2b ). A similar measurement was carried out for 2 ( Fig. 2c ) and the conductance histogram shows a peak located near 2.2×10 −5 G 0 ( Fig. 2d ), which is much smaller than the conductance of molecule 1 . This difference is expected because 2 has an extra 4-methylene-phenyl-1-ethynyl spacer between the coronene central block and the linker group, which disrupts the conjugation due to the presence of σ-bonds. The effect of linker group in the conductance of molecules has been observed in other systems [11] , [13] . Figure 2: Conductance of single HBC molecules. ( a ) Individual conductance traces of 1 . Observed plateaus (arrows) are due to the breakdown of molecule–electrode contacts. For comparison, control experiments carried out in the absence of molecules are also shown. ( b ) Conductance histogram constructed from thousands of individual conductance traces for 1 . ( c ) Individual conductance traces of 2 . ( d ) Conductance histogram constructed from thousands of individual conductance traces for 2 . Note that the large counts near the edges on both histogram plots ( b , d ) are due to background noises. Full size image We studied the gate effect of individual HBC molecules using the following procedures [14] . First, we moved the STM tip close to the substrate covered with a dilute layer of HBC molecules until the tunnelling current between the tip and the substrate reached a preset value. We then froze the tip position, and monitored the current continuously. During this process, the current frequently switched abruptly to a much higher value, and then back to the original value. This switching behaviour is due to the attachment/detachment of an HBC molecule to/from the STM tip through the amine or thiol linker group (blue line in Fig. 3a ) [15] . As a control experiment, we varied the tip–substrate distance, and observed the switching only when the tip–substrate distance was less than the length of the molecules. We carried out a further control experiment using a blank substrate and observed no switching in the tunnelling current. Finally, we point out that the conductance of the high current state agrees with the steps in the conductance traces and with peaks in the conductance histograms presented in Fig. 2 . Once a molecule was bridged between the substrate and tip electrodes, we swept the electrochemical gate voltage and recorded the source-drain current ( I sd ) as a function of gate voltage ( V g ) and time (red line, in Fig. 3a ). 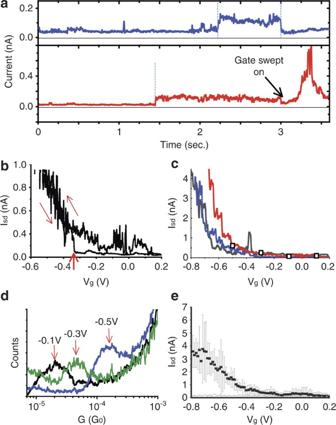Figure 3: Gate effect of single HBC molecule FET. (a) Formation and breakdown of single HBC molecule FETs (blue) are observed as current switching between two levels. The high-current level corresponds to electron transport through the molecule, and the low-current level is due to tunnelling through space. When a HBC molecule bridges the substrate and tip electrodes, applying an electrochemical gate causes a large change in transport current (red). Note that conductance reduces slightly immediately after starting gate sweep (gate on) to 0.2 V and progressively increases when it is swept back to −0.8 V (see curvesb, c, e). (b) A typical gate dependence of the source-drain current of a single molecule HBC FET device. The sudden decrease marked by a red arrow in the current during measurement is due to the breakdown of molecule–electrode contact. (c) Gate effect of three different HBC molecule FETs. The average gate dependence obtained from conductance histograms is shown as open squares. (d) Conductance histograms at different gate voltages. (e) Averaged source-drain current versus gate voltage (black dots) and variations (error bars). Open circles represent the source-drain current versus gate voltage of a tunnelling gap with no molecules present. All the results shown in this figure are from2. Figure 3: Gate effect of single HBC molecule FET. ( a ) Formation and breakdown of single HBC molecule FETs (blue) are observed as current switching between two levels. The high-current level corresponds to electron transport through the molecule, and the low-current level is due to tunnelling through space. When a HBC molecule bridges the substrate and tip electrodes, applying an electrochemical gate causes a large change in transport current (red). Note that conductance reduces slightly immediately after starting gate sweep (gate on) to 0.2 V and progressively increases when it is swept back to −0.8 V (see curves b, c, e ). ( b ) A typical gate dependence of the source-drain current of a single molecule HBC FET device. The sudden decrease marked by a red arrow in the current during measurement is due to the breakdown of molecule–electrode contact. ( c ) Gate effect of three different HBC molecule FETs. The average gate dependence obtained from conductance histograms is shown as open squares. ( d ) Conductance histograms at different gate voltages. ( e ) Averaged source-drain current versus gate voltage (black dots) and variations (error bars). Open circles represent the source-drain current versus gate voltage of a tunnelling gap with no molecules present. All the results shown in this figure are from 2 . Full size image Figure 3b is a typical I sd versus V g plot for 2 , showing an increase in current when the gate voltage sweeps towards negative values. We note that the sign convention of the electrochemical gate is the reverse of that used in solid-state semiconductor devices. It is interesting to point out here that the current drops suddenly back to the small tunnelling background level when the gate voltage sweeps back to approximately −0.35 V, indicating the breakdown of the molecule–electrode contact. This breakdown process was frequently observed in many I sd versus V g runs. Figure 3c displays several individual I sd versus V g traces. The current does not change much until the gate voltage lowers to −0.2 V, below which the current increases sharply, revealing n-type FET characteristics and implying electrons as the charged carriers. At more negative gate voltages than −0.8 V, the thiol-gold bond becomes unstable; hence it was set as the lower limit in I sd versus V g runs. The positive limit of the gate voltage was +0.5 V, which is determined by the stability of the gold electrode, and prevented us from observing p-type transport behaviour. We also studied the gate effect using the statistical analysis approach, which measured conductance histograms at different gate voltages. As shown in Figure 3d, the peak in the histogram for 1 shifts towards higher conductance values as gate voltage decreases. The source-drain current values determined from conductance at different gate voltages are plotted as open squares in Fig. 3c . There are some device-to-device variations, which are likely due to variations in the molecule–electrode contact geometry. This is evident from the broad peaks in the conductance histograms ( Figs 2 and 3d ). Figure 3e shows an I sd versus V g plot averaged over 50 devices. Despite the variations (error bars), the gate effect is repeatedly observed in all the devices. For comparison, the transport current through a tunnelling gap after the breakdown of an HBC molecule is also plotted as a function of gate voltage in Fig. 3e (open circles), which shows no gate dependence. We have also studied the gate effect on 1 , but the gate voltage that could be applied to the device was within a much smaller window because of the instability of the weaker amine–gold contact. The HOMO–LUMO gap of both molecules calculated using density functional theory and estimated from the optical absorption spectra is ∼ 3.2 eV (see Supplementary Information, sections 3 and 4 ). By adjusting the gate voltage, one can move the Fermi levels of the source and drain electrodes towards the HOMO or LUMO levels. However, cyclic voltammetry measurements of the HBC self-assembled monolayer on gold electrodes within the gate voltage window used in I sd versus V g curves did not show any redox peaks that could be associated with the electron transfer between the molecules and electrodes. This indicates that the Fermi energy levels could not be aligned to either the LUMO or the HOMO level, preventing us from achieving transport through the LUMO or HOMO. It also indicates electron tunnelling as the transport mechanism in these molecules. To elucidate the transport mechanism, we carried out temperature-dependent transport measurements on single-molecule junctions by recording conductance histograms at different temperatures (see Fig. 4a ). To simplify the experimental set up, measurements were taken without electrochemical control in an inert organic environment (mesitylene). We found that the conductance values of HBC molecules are insensitive to temperature within the experimental uncertainty over the experimentally accessible temperature window (−5 to 40°C) (see Fig. 4b ). This observation strongly suggests electron tunnelling as the dominant transport mechanism in these single-molecule junctions, which is inconsistent with the alignment of the molecular HOMO/LUMO levels with the electrode Fermi level. We believe then that the large increase in transport current at negative gate voltages is due to the tail of the resonant tunnelling through the LUMO of the molecules. Full resonance condition cannot be reached because of the instability of the molecule–electrode contact at more negative gate voltages. 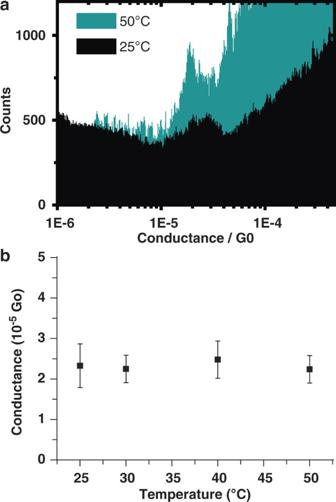Figure 4: Temperature dependence transport measurements. (a) Conductance histograms of molecule1at two different temperatures in mesitylene. Arrow marks the position of the peaks. (b) Conductance versus temperature for molecule1collected from the histograms. Figure 4: Temperature dependence transport measurements. ( a ) Conductance histograms of molecule 1 at two different temperatures in mesitylene. Arrow marks the position of the peaks. ( b ) Conductance versus temperature for molecule 1 collected from the histograms. Full size image The largest on/off ratio achieved for these molecular systems is about 50, which is larger than most graphene FETs fabricated using the top-down approach [16] . This ratio could be increased using a more stable electrode–molecule contact. An alternative way to improve the on-off ratio is to increase the length of the molecules. Recently, Perez-Jimenez and Sancho-Garcia [17] have shown that the HOMO–LUMO gap of large polycyclic aromatic molecules is inversely proportional to the molecular length. The 13-ring coronene devices exhibit a gate dependence that resembles graphene nanoribbons, but they are still different from the large graphene sheets that have the characteristic band structure. By increasing the size of the molecule, one may study and understand the transition from discrete molecular energy levels to the band structure. Larger molecules would also make the device fabrication more compatible with conventional fabrication techniques, and help to bridge the technical gap between the bottom-up and the conventional top-down approach. This bottom-up approach points to a new avenue for the fabrication of nanographene electronic devices and, more important, for the understanding of the size dependence and exploration of the rich properties of the important family of carbon materials at the smallest dimensions. Synthesis Synthesis procedures of 1 and 2 were based on the protocols established for the synthesis of other derivatives of HBC (see Supplementary Information ). The key difference is the introduction of the linker groups needed to form reliable and efficient coupling between electrodes and molecules. In the case of 1 , major synthetic effort was made to attach the two terminal amine groups directly onto the coronene scaffold, enabling the construction of a simple break junction composed of only the graphene component of interest. For 2 , synthesis was based on metal-catalysed cross-coupling with para-dibromo-substituted HBC. This approach offers the opportunity to attach thiol groups to HBC through additional spacers, so that the distance and conjugation between the coronene core and anchor group can be controlled. The details of the modified synthesis, purification and structural characterization are detailed in Supporting Information . Transport measurements Each break junction experiment comprised a total of 1000–2500 conductance versus distance traces collected at a given source-drain voltage (tip–substrate bias) and electrochemical gate voltage. The pulling rates were 20–40 nm s −1 . The gate effect of individual devices was carried out with the same setup as the STM break junction but using the following procedure. First, we started the experiment with a low set-point current to ensure the tip–substrate distance that was larger than the molecular length. In this case, no molecules could bridge between the tip and substrate electrodes, and the tunnelling through the space between the tip and the substrate dominated the current. The tip–substrate distance was then reduced below the molecular length to allow the individual HBC molecules to bridge across the tip and substrate electrodes, which led to large stepwise switching events in the current. The gate effect was studied by sweeping the gate voltage when the current jumped to the high current state. STM tips were prepared by freshly cutting gold wires (99.998%) with a diameter of 0.25 mm. Gold substrates were prepared by thermally evaporating 130 nm gold (99.999%) on freshly cleaved mica in a ultrahigh vacuum chamber. Before each experiment, a substrate was annealed with an hydrogen flame for ∼ 1 min, and then immediately immersed in mesitylene or ionic liquid, 1-butyl-3-methylimida-zolium hexafluorophosphate. The electrochemical gate experiment was carried out using a sample cell made of Teflon using the ionic liquid as electrolyte. The cell was cleaned in boiling Piranha (98% H 2 SO 4 : 30% H 2 O 2 =3:1, V/V) for ∼ 30 mins, and then thoroughly rinsed in boiling water (18 MΩ, Nanopure system fed with campus distilled water) three times. A freshly cut silver wire was used as quasi reference and a platinum wire as the counter electrode, and the potentials of the tip and substrate electrodes were controlled using a biopotentiostat (Molecular Imaging). For 1 , the conductance traces were clean and the conductance histogram at each gate voltage and bias was constructed using all the curves with no selection. For 2 , however, the individual traces are noisier, which is at least partially due to the smaller current (lower conductance), compared with 1 . In the last case, to construct the conductance histogram, extremely noisy conductance traces are removed. Conductance measurements at different temperatures were determined for 2 in mesitylene. The temperature of gold substrates was controlled by a Peltier stage (Molecular Imaging) within the −5 to 40°C range and by a resistive stage for higher temperatures. How to cite this article: Diez-Perez, I. et al . Gate-controlled electron transport in coronenes as a bottom-up approach towards graphene transistors. Nat. Commun. 1:31 doi: 10.1038/ncomms1029 (2010).